Gαsregulates the post-endocytic sorting of G protein-coupled receptors The role of Gα s in G protein-coupled receptor (GPCR) signalling at the cell surface is well established. Recent evidence has revealed the presence of Gα s on endosomes and its capacity to elicit GPCR-promoted signalling from this intracellular compartment. Here, we report an unconventional role for Gα s in the endocytic sorting of GPCRs to lysosomes. Cellular depletion of Gα s specifically delays the lysosomal degradation of GPCRs by disrupting the transfer of GPCRs into the intraluminal vesicles (ILVs) of multivesicular bodies. We show that Gα s interacts with GPCR-associated binding protein-1 (GASP1) and dysbindin, two key proteins that serve as linkers between GPCRs and the endosomal-sorting complex required for transport (ESCRT) machinery involved in receptor sorting into ILVs. Our findings reveal that Gα s plays a role in both GPCR signalling and trafficking pathways, providing another piece in the intertwining molecular network between these processes. Heterotrimeric G proteins, which are composed of α, β and γ subunits, transduce extracellular signals from G protein-coupled receptors (GPCRs) to intracellular downstream effector proteins. In the conventional G protein-signalling paradigm, the G protein localizes to the cytoplasmic surface of the plasma membrane (PM), where after activation by an agonist-bound GPCR, the guanosine triphosphate (GTP)-bound Gα and free Gβγ bind to and regulate a number of well-studied effectors, including adenylyl cyclase, phospholipase Cβ and ion channels [1] . However, over the past decade, research has established that G proteins also have non-canonical roles in the cell, such as in regulating novel effectors [2] , [3] , [4] , undergoing GPCR-independent activation [5] and acting on organelles [2] , [3] , [4] , [5] , [6] . Indeed, in addition to localizing to the PM, heterotrimeric G proteins are found on the membranes of intracellular compartments along both the endocytic and secretory pathways, where mounting evidence suggest they play several roles in membrane trafficking [5] , [7] , [8] , [9] , [10] . Longstanding evidence have suggested that Gα s is involved in endosomal functions [11] , [12] , [13] , [14] . Several recent studies have confirmed that Gα s is present on endosomes and has non-conventional roles in endosomal receptor signalling and trafficking [15] , [16] , [17] , [18] , [19] . The ability of Gα s to be activated and signal from this intracellular compartment was recently observed following the internalization of vasopressin type 2 receptor, parathyroid hormone receptor (PTHR) and β2-adrenergic receptor (β2AR), all of which are Gα s -coupled GPCRs [15] , [16] , [20] . Gα s also regulates the endosomal sorting and downregulation of epidermal growth factor receptor (EGFR), a single transmembrane-spanning receptor [18] . However, the role of Gα s in the endosomal sorting of other receptors, its precise molecular mechanism and the role of its activation status (guanosine diphosphate (GDP)/GTP forms) in this trafficking step remain undefined. GPCR activity is tightly controlled by endocytic pathway. Ligand-induced internalization drives GPCRs into early endosomes, where they are either recycled back to the PM for another round of activation or sorted to the lysosomes for degradation, producing a prolonged attenuation of cellular signalling. Lysosomal sorting of GPCRs occurs via a highly conserved mechanism requiring recognition by the endosomal-sorting complex required for transport (ESCRT), which sorts receptors into the intraluminal vesicles (ILVs) of multivesicular bodies (MVBs), leading to a point of no return for complete degradation in lysosomes [21] , [22] . Certain GPCRs are ubiquitinated, which regulates their direct interaction with the hepatocyte growth factor regulated tyrosine kinase substrate (HRS) component of the ESCRT machinery [23] , [24] , [25] . However, several GPCRs are sorted by the ESCRT machinery independent of ubiquitination [22] , [26] , [27] . Recent work has demonstrated that GPCR-associated binding protein-1 (GASP-1) and dysbindin link a subset of GPCRs to the ESCRT machinery. GASP-1 binds to the carboxyl-termini of several GPCRs and targets them to the lysosomal pathway [28] , [29] , [30] . Dysbindin, a cytoplasmic protein that functions in the biogenesis of specialized lysosome-related organelles, has recently been shown to promote the lysosomal sorting of δ-opioid receptor (DOP) and dopamine 2 receptor (D2R) and is thought to link GASP-1 to the HRS component of the ESCRT machinery [31] . A mechanistic understanding of GPCR endosomal sorting is only beginning to emerge. In the present study, we investigated whether Gα s is involved in the regulation of the endocytic sorting of GPCRs. Our results showed that Gα s is critical for sorting GPCRs into the ILVs of MVBs through interactions with GASP-1, dysbindin and the ESCRT machinery. These interactions were independent of Gα s GTPase activity. This study defines a novel regulatory role for Gα s in the post-endocytic sorting and downregulation of GPCRs. Gα s is required for the degradation of a subset of GPCRs Gα s can localize to endosomes and participate in EGFR trafficking and signalling [17] , [18] , [19] . Because GPCRs are specifically sorted in endosomes, we investigated whether Gα s is involved in the endocytic trafficking of these receptors. We first analysed the impact of Gα s depletion on the basal levels of various GPCRs that are either sorted in the lysosomes (chemokine receptor type 4 (CXCR4), DOP, D2R and angiotensin 1 receptor (AT1R)) or recycled to the PM (β2AR, μ-opioid receptor (MOP) and dopamine 1 receptor (D1R)) ( Fig. 1a ). Tagged GPCRs were expressed in HEK293 cells transfected with control or Gα s short interfering RNA (siRNA), and western blot (WB) analysis revealed that the expression levels of CXCR4, DOP, D2R and AT1R were increased in Gα s -depleted cells, whereas the β2AR, MOP and D1R levels were unaffected. The quantification analysis confirmed the higher levels of lysosome-targeted GPCRs in steady-state cells transfected with Gα s siRNA ( Fig. 1b ), suggesting that the basal turnover of these receptors was delayed by Gα s knockdown. This result was confirmed with endogenous CXCR4. Gα s depletion led to a significant increase in the steady-state expression of endogenous CXCR4 in HeLa cells, a cell line that expresses high levels of endogenous CXCR4 and Gα s ( Supplementary Fig. 1a ), suggesting that Gα s similarly regulated the basal turnover of an endogenous GPCR. The specificity of the effect of Gα s on GPCR levels was validated in two different manners. First, the depletion of Gα i3 and Gβ 1 did not affect the basal levels of haemagglutinin (HA)–CXCR4 or HA–DOP ( Supplementary Fig. 1b ). Second, after reintroducing Gα s into Gα s -depleted cells with siRNA-resistant forms of the short and long variants of human Gα s , the basal levels of HA–CXCR4 and HA–DOP were similar to or lower than those in the control cells ( Supplementary Fig. 1c ), confirming a specific role for Gα s in influencing the levels of these particular GPCRs. Interestingly, all of the GPCRs that were affected by Gα s depletion are not coupled to Gα s in their conventional signalling pathways. Indeed, DOP, CXCR4 and D2R are coupled to Gα i/o (refs 32 , 33 , 34 ), and AT1R is coupled to Gα i/q (ref. 35 ). 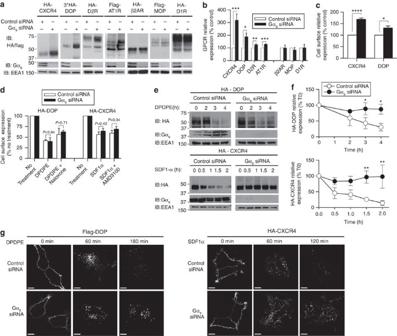Figure 1: Gαsknockdown delays GPCR degradation. (a) Representative immunoblots (IB) of the steady-state levels of various tagged GPCRs transiently expressed in HEK293 cells treated with control or GαssiRNA. EEA1, loading control. (b) Quantification of the GPCR expression ina. The data are presented as the percentage of GPCR expression compared with control cells. GPCRs in the left part of the histogram have a higher propensity to downregulate rather than to recycle and are not coupled to Gαsfor signalling. (c) Quantification of the cell-surface expression of HA–DOP and HA–CXCR4 in HEK293 cells treated with control or GαssiRNA. ELISAs were performed to measure cell-surface receptor expression. (d) Quantification of the internalization and recycling rates of HA–DOP and HA–CXCR4 in cells treated with control or GαssiRNA. ELISAs were performed to measure cell-surface receptor levels in HEK293 cells that were untreated, treated with agonist (5 μM DPDPE or 100 nM SDF1-α) for 30 min (to measure internalization) or treated with agonist followed by antagonist (10 μM naloxone or AMD3100) for 60 min (to measure recycling). Data are presented as the percentage of GPCR expression compared with untreated cells. (e) Representative immunoblots of the kinetics of Flag–DOP and HA–CXCR4 degradation following agonist stimulation in control or Gαs-depleted HEK293 cells. Different film exposures were used for the control and GαssiRNA blots to better show the differences in the degradation kinetics. (f) Quantification of the GPCR expression ine. Data are presented as the percentage of GPCR expression compared with unstimulated cells (T0). (g) Immunofluorescence analysis of Flag–DOP and HA–CXCR4 internalization in HEK293 cells transfected with control or GαssiRNA. Cell-surface GPCRs were labelled with anti-Flag or anti-HA at 4 °C before incubation at 37 °C in the presence of agonists. At the indicated times, cells were processed for confocal microscopy analysis. For each time point, images were acquired using identical instrument settings. Scale bars, 10 μm. The data inb–dandfare presented as the mean±s.e.m. of ≥3 independent experiments. Statistical analysis was performed using the Student’st-test. *P≤0.05, **P≤0.01, ***P≤0.001, ****P≤0.0001. Figure 1: Gα s knockdown delays GPCR degradation. ( a ) Representative immunoblots (IB) of the steady-state levels of various tagged GPCRs transiently expressed in HEK293 cells treated with control or Gα s siRNA. EEA1, loading control. ( b ) Quantification of the GPCR expression in a . The data are presented as the percentage of GPCR expression compared with control cells. GPCRs in the left part of the histogram have a higher propensity to downregulate rather than to recycle and are not coupled to Gα s for signalling. ( c ) Quantification of the cell-surface expression of HA–DOP and HA–CXCR4 in HEK293 cells treated with control or Gα s siRNA. ELISAs were performed to measure cell-surface receptor expression. ( d ) Quantification of the internalization and recycling rates of HA–DOP and HA–CXCR4 in cells treated with control or Gα s siRNA. ELISAs were performed to measure cell-surface receptor levels in HEK293 cells that were untreated, treated with agonist (5 μM DPDPE or 100 nM SDF1-α) for 30 min (to measure internalization) or treated with agonist followed by antagonist (10 μM naloxone or AMD3100) for 60 min (to measure recycling). Data are presented as the percentage of GPCR expression compared with untreated cells. ( e ) Representative immunoblots of the kinetics of Flag–DOP and HA–CXCR4 degradation following agonist stimulation in control or Gα s -depleted HEK293 cells. Different film exposures were used for the control and Gα s siRNA blots to better show the differences in the degradation kinetics. ( f ) Quantification of the GPCR expression in e . Data are presented as the percentage of GPCR expression compared with unstimulated cells (T0). ( g ) Immunofluorescence analysis of Flag–DOP and HA–CXCR4 internalization in HEK293 cells transfected with control or Gα s siRNA. Cell-surface GPCRs were labelled with anti-Flag or anti-HA at 4 °C before incubation at 37 °C in the presence of agonists. At the indicated times, cells were processed for confocal microscopy analysis. For each time point, images were acquired using identical instrument settings. Scale bars, 10 μm. The data in b – d and f are presented as the mean±s.e.m. of ≥3 independent experiments. Statistical analysis was performed using the Student’s t- test. * P ≤0.05, ** P ≤0.01, *** P ≤0.001, **** P ≤0.0001. Full size image To determine whether the upregulated GPCRs in steady-state Gα s -depleted cells localized to the PM, we measured the surface levels of these receptors as a function of Gα s expression. We focused on CXCR4 and DOP because these two GPCRs were most affected by Gα s depletion ( Fig. 1a,b ). A cell surface enzyme-linked immunosorbent assay (ELISA) demonstrated that the cell surface expression of HA–DOP and HA–CXCR4 was significantly increased in Gα s -depleted HEK293 cells ( Fig. 1c ). As the amount of a cell surface receptor is partly a function of the rate of receptor internalization and recycling, we next examined the effect of Gα s depletion on the internalization and recycling of HA-tagged CXCR4 and DOP by ELISA ( Fig. 1d ). No significant differences were observed between control and Gα s -depleted cells ( Fig. 1d ), indicating that Gα s depletion had no effect on the internalization and recycling of these GPCRs and suggesting that Gα s instead affected their constitutive trafficking and degradation. Accordingly, immunofluorescence (IF) microscopy analysis of the steady-state distribution of HA-tagged CXCR4 in HEK293 cells showed an accumulation of CXCR4 in intracellular vesicles in Gα s -depleted cells, whereas CXCR4 predominantly localized to the PM in control cells ( Supplementary Fig. 1d ). Together, these results suggested that the increased steady-state levels of CXCR4 and DOP in Gα s -depleted cells were owing to the involvement of Gα s in the constitutive trafficking and turnover of these receptors. We next investigated whether Gα s depletion affected ligand-mediated GPCR trafficking and turnover. We assessed the effect of Gα s depletion on the kinetics of the ligand-dependent degradation of CXCR4 and DOP. Cells transiently overexpressing HA-tagged CXCR4 or DOP and transfected with control or Gα s siRNA were treated with agonists in the presence of cycloheximide (to block de novo protein synthesis) for the indicated time, and GPCR abundance was monitored by WB and quantified ( Fig. 1e ). In cells transfected with control siRNA, >70% of the DOP and CXCR4 receptors were degraded after stimulation for 4 h or 2 h, respectively, whereas in cells transfected with Gα s siRNA, <20% of the receptors were degraded ( Fig. 1f ). The significantly reduced rate of receptor degradation in agonist-stimulated, Gα s -depleted cells indicated a requirement for Gα s in the establishment of ligand-mediated GPCR turnover, suggesting that proper GPCR trafficking and sorting is dependent on Gα s . IF microscopy was utilized to evaluate the effects of Gα s depletion on the endocytosis and degradation of cell-surface-labelled DOP and CXCR4 ( Fig. 1g ). After agonist stimulation for 60 min, the amount of DOP and CXCR4 that was internalized into vesicles was similar in control and Gα s -depleted cells, confirming that Gα s depletion did not impair GPCR internalization. However, after longer agonist treatments (120 or 180 min), cell-surface-labelled DOP and CXCR4 were mostly degraded in control cells, but remained in intracellular vesicles in Gα s -depleted cells ( Fig. 1g ). Together, these results suggested that the decreased degradation of DOP and CXCR4 in Gα s -depleted cells was due to retention in intracellular compartments. Gα s promotes GPCR sorting in the ILVs of MVBs To identify the intracellular compartment in which DOP and CXCR4 were retained in Gα s -depleted cells, we examined the distribution of internalized HA-tagged DOP and CXCR4 in control and Gα s siRNA-treated cells ( Fig. 2a ). After 15 min of agonist stimulation, cell-surface-labelled DOP and CXCR4 colocalized with the early endosomal marker EEA1 in both control and Gα s -depleted cells. After 120 or 180 min of agonist stimulation, DOP and CXCR4 showed little colocalization with EEA1 in control cells, consistent with receptor trafficking out of the early endosome to the late endosome/lysosomes. In contrast, DOP and CXCR4 exhibited robust colocalization with EEA1 in Gα s siRNA-treated cells at this later time point. The quantitative analysis confirmed a significant increase in the colocalization of DOP and CXCR4 with EEA1-positive endosomes in Gα s -depleted cells compared with control cells ( Fig. 2b ). These results suggested that DOP and CXCR4 were trapped in early endosomes in the absence of Gα s . 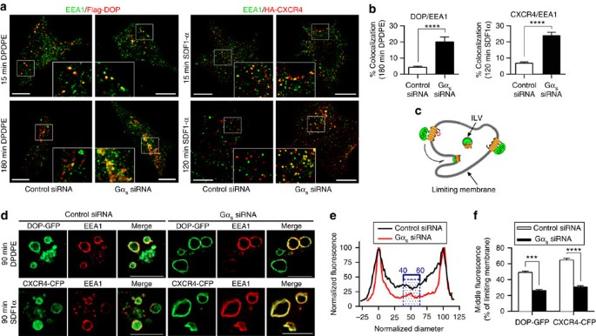Figure 2: Gαsknockdown alters the transfer of GPCRs to the ILVs of MVBs. (a) Gαsdepletion prolonged the presence of internalized Flag–DOP and HA–CXCR4 in early endosomes. Confocal microscopy images comparing the distribution of the early endosome marker EEA1 and the cell-surface-labelled Flag–DOP and HA–CXCR4 in control or Gαs-depleted HEK293 cells treated with agonist for 15, 120 or 180 min. Scale bars, 10 μm. The images were acquired at different laser and photomultiplier (PMT) settings to enable the detection of the GPCRs at each time point and to compare their localization with EEA1. (b) Quantification of the degree of overlap between EEA1 and HA–CXCR4 or Flag–DOP in cells treated with control or GαssiRNA. (c) Diagram illustrating the distribution of a GPCR with a C-terminal GFP tag on the outer membrane of an endosome and in ILVs. (d) Gαsdepletion prevented the redistribution of DOP–GFP and CXCR4–CFP from the endosome-limiting membrane to the ILVs. Representative optical sections depict endosomes in control and Gαs-depleted HEK293 cells co-transfected with DOP–GFP or CXCR4–CFP along with Rab5-Q79L (to create enlarged endosomes) and treated with agonist for 90 min. Cells were fixed and processed for confocal microscopy. Scale bars, 10 μm. (e) Representative line scan analysis to quantify GPCR–GFP localization to the ILVs of endosomes. The normalized diameter represents the diameter of the endosome, where 0 and 100 correspond to the pixel distances with the first and second maximum pixel intensities, signifying the limiting membranes of the endosomes. The black and red traces represent the normalized fluorescence pixel intensity measured across the endosomes in control and Gαs-depleted cells, respectively, with the maximum pixel intensity across the line normalized to 100. The hatched box highlights the normalized fluorescence values of pixels from 40 to 60% of the normalized diameter that were used to determine the mean intraluminal fluorescence for each endosome. (f) Compiled results of the line scan analysis for DOP–GFP and CXCR4–CFP. The data inbandfare presented as the mean±s.e.m. of n≥100 cells or endosomes, respectively, from three independent experiments. Statistical analysis was performed using the Student’st-test. ***P<0.001, ****P≤0.0001. Figure 2: Gα s knockdown alters the transfer of GPCRs to the ILVs of MVBs. ( a ) Gα s depletion prolonged the presence of internalized Flag–DOP and HA–CXCR4 in early endosomes. Confocal microscopy images comparing the distribution of the early endosome marker EEA1 and the cell-surface-labelled Flag–DOP and HA–CXCR4 in control or Gα s -depleted HEK293 cells treated with agonist for 15, 120 or 180 min. Scale bars, 10 μm. The images were acquired at different laser and photomultiplier (PMT) settings to enable the detection of the GPCRs at each time point and to compare their localization with EEA1. ( b ) Quantification of the degree of overlap between EEA1 and HA–CXCR4 or Flag–DOP in cells treated with control or Gα s siRNA. ( c ) Diagram illustrating the distribution of a GPCR with a C-terminal GFP tag on the outer membrane of an endosome and in ILVs. ( d ) Gα s depletion prevented the redistribution of DOP–GFP and CXCR4–CFP from the endosome-limiting membrane to the ILVs. Representative optical sections depict endosomes in control and Gα s -depleted HEK293 cells co-transfected with DOP–GFP or CXCR4–CFP along with Rab5-Q79L (to create enlarged endosomes) and treated with agonist for 90 min. Cells were fixed and processed for confocal microscopy. Scale bars, 10 μm. ( e ) Representative line scan analysis to quantify GPCR–GFP localization to the ILVs of endosomes. The normalized diameter represents the diameter of the endosome, where 0 and 100 correspond to the pixel distances with the first and second maximum pixel intensities, signifying the limiting membranes of the endosomes. The black and red traces represent the normalized fluorescence pixel intensity measured across the endosomes in control and Gα s -depleted cells, respectively, with the maximum pixel intensity across the line normalized to 100. The hatched box highlights the normalized fluorescence values of pixels from 40 to 60% of the normalized diameter that were used to determine the mean intraluminal fluorescence for each endosome. ( f ) Compiled results of the line scan analysis for DOP–GFP and CXCR4–CFP. The data in b and f are presented as the mean±s.e.m. of n≥100 cells or endosomes, respectively, from three independent experiments. Statistical analysis was performed using the Student’s t- test. *** P <0.001, **** P ≤0.0001. Full size image Following internalization in early endosomes, GPCRs destined for lysosomal degradation, such as DOP and CXCR4, are transferred from the endosome-limiting membranes to the ILVs of MVBs. We thus examined whether Gα s altered the sorting of GPCRs into ILVs. DOP and CXCR4 were tagged at their C terminus with green fluorescent protein (GFP) (DOP–GFP) or cyan fluorescent protein (CFP) (CXCR4–CFP), and were co-expressed with constitutively active Rab5 (Rab5-Q79L) to create enlarged endosomes and to facilitate the detection of these GPCRs on the limiting and intraluminal membranes of MVBs ( Fig. 2c ). Confocal microscopy analysis of control cells stimulated with agonist for 90 min showed the presence of DOP–GFP and CXCR4–CFP in both the limiting membranes and the ILVs of enlarged endosomes labelled with EEA1 ( Fig. 2d ). In contrast, in Gα s -depleted cells, DOP–GFP and CXCR4–CFP localized predominantly to the limiting membranes of enlarged endosomes, with most endosomes exhibiting little intraluminal fluorescence ( Fig. 2d ). The GPCR distribution across the endosomes was quantified by line scan analysis of confocal cross-sections as previously described [36] . A representative line scan analysis of an endosome is shown in Fig. 2e . The peaks indicate the limiting membrane, and the hatched box indicates the central region of the endosome lumen. An analysis of >100 endosomes from multiple cells and experiments revealed a 50% reduction in both DOP–GFP and CXCR4–CFP in the endosomal lumen in Gα s -depleted cells compared with control cells ( Fig. 2f ). Taken together, these results indicated that Gα s plays a crucial role in the sorting of GPCRs in the ILVs of MVBs for subsequent lysosomal degradation. Gα s is a component of the GPCR endosomal-sorting machinery To decipher the molecular mechanism by which Gα s regulates GPCR degradation, we next examined whether Gα s associates with the core machinery that mediates sorting into the ILVs of MVBs. ESCRT molecules, including HRS (ESCRT-0), are central players in the endosomal sorting of GPCRs [25] , [27] . HRS can either function directly by interacting with a ubiquitinated GPCR (such as CXCR4) [25] or indirectly by interacting with the accessory proteins GASP-1 and dysbindin, which are part of an alternate connectivity network linking particular GPCRs (such as DOP and D2R) to the ESCRT machinery [28] , [29] , [30] , [31] . To determine whether Gα s associates with these endocytic sorting components, HEK293 cells were transiently transfected with GFP or Gα s –GFP together with untagged HRS, Myc-tagged dysbindin or Cherry-tagged GASP-1, and immunoprecipitations were performed with an anti-GFP antibody. Gα s –GFP interacted with HRS, dysbindin and GASP-1 ( Fig. 3a ), suggesting that Gα s is part of this sorting machinery. These interactions were specific for Gα s , as the Gα proteins Gα i3 , Gα q and Gα z did not precipitate HRS, dysbindin or GASP-1 ( Supplementary Fig. 2a ). 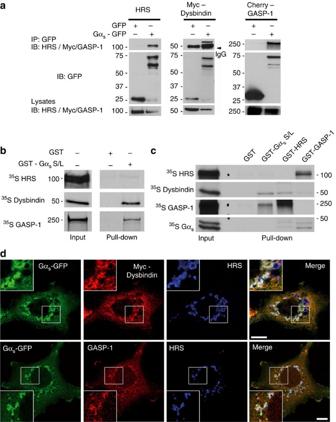Figure 3: Gαsinteracts and colocalizes with the GASP-1–dysbindin–HRS endosomal-sorting machinery. (a) Immunoprecipitation of Gαs–GFP with HRS, Myc–dysbindin and Cherry–GASP-1. Lysates from HEK293 cells transiently transfected with GFP or Gαs–GFP along with HRS, Myc–dysbindin or Cherry–GASP-1 were immunoprecipitated (IP) with anti-GFP and immunoblotted (IB) using the indicated antibody. (b) GST pull-down experiment demonstrating that dysbindin and GASP-1, but not HRS, interact directly with Gαs.In vitrotranslated35S-labelled dysbindin and GASP-1 bound to GST–Gαs(short (S) and long (L) forms) but not to GST.35S-labelled HRS did not bind to GST–Gαs. Bound proteins were separated by SDS–PAGE and detected by autoradiography. (c) GST pull-down experiments to define the protein complex containing GASP-1, dysbindin, HRS and Gαs.In vitrotranslated35S-labelled HRS, dysbindin, GASP-1 and Gαswere incubated with GST alone, GST–Gαs, GST–HRS or GST–GASP-1. The samples were analysed as inb. (d) Immunofluorescence analysis of COS7 cells transfected with Gαs–GFP and Myc–dysbindin or Cherry–GASP-1. The cells were fixed, labelled with anti-GFP, anti-HRS and anti-Myc or anti-Cherry and then processed for confocal microscopy. The overexpression of Gαstogether with dysbindin or GASP-1 promoted the formation of clustered and enlarged endosomes. Merged images illustrate the colocalization of Gαs, endogenous HRS and dysbindin or GASP-1 on endosomes. Scale bars, 10 μm. Figure 3: Gα s interacts and colocalizes with the GASP-1–dysbindin–HRS endosomal-sorting machinery. ( a ) Immunoprecipitation of Gα s –GFP with HRS, Myc–dysbindin and Cherry–GASP-1. Lysates from HEK293 cells transiently transfected with GFP or Gα s –GFP along with HRS, Myc–dysbindin or Cherry–GASP-1 were immunoprecipitated (IP) with anti-GFP and immunoblotted (IB) using the indicated antibody. ( b ) GST pull-down experiment demonstrating that dysbindin and GASP-1, but not HRS, interact directly with Gα s . In vitro translated 35 S-labelled dysbindin and GASP-1 bound to GST–Gα s (short (S) and long (L) forms) but not to GST. 35 S-labelled HRS did not bind to GST–Gα s . Bound proteins were separated by SDS–PAGE and detected by autoradiography. ( c ) GST pull-down experiments to define the protein complex containing GASP-1, dysbindin, HRS and Gα s . In vitro translated 35 S-labelled HRS, dysbindin, GASP-1 and Gα s were incubated with GST alone, GST–Gα s , GST–HRS or GST–GASP-1. The samples were analysed as in b . ( d ) Immunofluorescence analysis of COS7 cells transfected with Gα s –GFP and Myc–dysbindin or Cherry–GASP-1. The cells were fixed, labelled with anti-GFP, anti-HRS and anti-Myc or anti-Cherry and then processed for confocal microscopy. The overexpression of Gα s together with dysbindin or GASP-1 promoted the formation of clustered and enlarged endosomes. Merged images illustrate the colocalization of Gα s , endogenous HRS and dysbindin or GASP-1 on endosomes. Scale bars, 10 μm. Full size image We next examined whether the interactions between Gα s and the sorting machinery components are direct. 35 S-labelled, in vitro -translated GASP-1, dysbindin or HRS was incubated with glutathione beads coated with glutathione S -transferase (GST) alone or with the short and long forms of Gα s fused to GST (GST–Gα s S/L). As shown in Fig. 3b , GST–Gα s bound to dysbindin and GASP-1, but not HRS, suggesting that Gα s bound directly to GASP-1 and dysbindin but required intermediate proteins to interact with HRS. Interestingly, dysbindin was identified by yeast two-hybrid as an interacting partner of HRS [37] , suggesting that dysbindin could be the link between Gα s and HRS. However, direct interactions between dysbindin and HRS or between dysbindin and GASP-1 have not been confirmed. To better define the complex containing GASP-1, dysbindin, HRS and Gα s , we generated GST–HRS and GST–GASP-1 and examined their interaction with 35 S-labelled, in vitro -translated Gα s, GASP-1, dysbindin or HRS ( Fig. 3c ). We confirmed that dysbindin interacted directly with HRS, and that Gα s interacted directly with GASP-1 but not with HRS. GASP-1 also interacted directly with HRS, but not with dysbindin. These results indicated that, although dysbindin and GASP-1 do not interact, they provide links between Gα s and HRS. We next investigated the intracellular localization of this protein complex. Gα s has been shown to localize with HRS on early endosomes [18] . To determine whether dysbindin and GASP-1 were present with Gα s on HRS-labelled endosomes, we performed immunofluorescent confocal microscopy on COS7 cells co-expressing Gα s –GFP and Myc–dysbindin or Cherry–GASP-1 ( Fig. 3d ). Myc–dysbindin had a largely diffuse cytoplasmic distribution, but a fraction colocalized with Gα s –GFP on HRS-positive endosomes. Similarly, Cherry–GASP-1 was mainly distributed throughout the cytoplasm but also colocalized with Gα s –GFP and endogenous HRS on sorting endosomes. Interestingly, the overexpression of Gα s together with either dysbindin or GASP-1 altered the morphology of the early endosomes, as previously reported for overexpressed HRS [38] , [39] , [40] . Taken together, these data suggested that the components of this sorting complex localize together on early endosomes and could facilitate the sorting of GPCRs into the degradative pathway. In agreement with this hypothesis, we confirmed that internalized HA–DOP and HA–CXCR4 colocalized with Gα s on early endosomes ( Supplementary Fig. 3 ). Gα s activation state does not alter GPCR endosomal sorting To determine whether the effect of Gα s on GPCR degradation depended on the GTPase activity of Gα s , we investigated whether the interaction of Gα s with the sorting components dysbindin, GASP-1 and HRS depended on the activation state of Gα s . Purified GST–Gα s or GST alone preloaded with GDP (to mimic the inactive state) or GDP/AlF 4 − or GTPγS (to mimic the active state) was incubated with 35 S-labelled, in vitro -translated GASP-1, dysbindin or HRS, and protein binding was analysed ( Fig. 4a ). Inactive and active GST–Gα s bound dysbindin and GASP-1 at similar levels and did not bind HRS, suggesting that the Gα s activation state did not influence these interactions. These results were confirmed using HEK293 cell lysates overexpressing Myc–dysbindin, Cherry–GASP-1 or untagged HRS ( Fig. 4b ). Again, the GST–Gα s interactions with dysbindin, GASP-1 and HRS were independent of the activation state of Gα s . The small differences that were observed were not reproducible. The same results were obtained with immunoprecipitation assays using Gα s –GFP mutants mimicking active or inactive Gα s [41] , [42] , [43] ( Supplementary Fig. 2b ), indicating that the Gα s activation state did not influence its interactions with GASP-1, dysbindin and HRS. 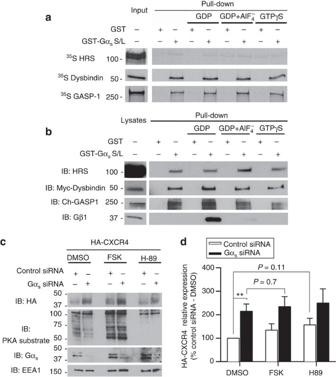Figure 4: The interaction of Gαswith the GPCR endosomal-sorting machinery is independent of the activation status of Gαs. (a)In vitroGST pull-down experiment showing that the Gαsactivation state did not influence its direct interactions with HRS, dysbindin and GASP-1.In vitrotranslated35S-labelled HRS, dysbindin and GASP-1 were incubated with GST alone or GST–Gαspreloaded with GDP (to mimic the inactive state) or GDP/AlF4−or GTPγS (to mimic the active state). Bound proteins were separated by SDS–PAGE and detected by autoradiography. (b) GST pull-down experiment in cell lysates demonstrating that the interactions between overexpressed dysbindin, GASP-1 and HRS were independent of the GST–Gαsactivation state. Lysates from HEK293 cells transiently transfected with HRS, Myc–dysbindin or Cherry–GASP-1 were incubated with GST alone, inactive GST–Gαs–GDP or active GST–Gαs–GDP/AlF4−or GTPγS (as described ina). Bound proteins were analysed by immunoblotting (IB) for HRS, Myc (dysbindin) and Cherry (GASP-1). The interaction with Gβ1 served as a control to confirm the activation state of GST–Gαsbecause Gβ1 only binds to inactive Gαs. This control was included in each experiment ina,b. (c) The downstream effectors of Gαswere not involved in CXCR4 downregulation. Control and Gαs-depleted HEK293 cells expressing HA–CXCR4 were treated for 8 h with vehicle (DMSO), 10 μM forskolin (an adenylyl cyclase activator) or 10 μM H89 (a PKA inhibitor). The steady-state levels of HA–CXCR4 were analysed by immunoblotting using the indicated antibody. (d) Quantification of the HA–CXCR4 levels inc. The data are presented as the percentage of HA–CXCR4 compared with control siRNA cells treated with DMSO. The data are presented as the mean±s.e.m. of ≥3 independent experiments and statistical analysis was performed using the Student’st-test. **P≤0.01. Figure 4: The interaction of Gα s with the GPCR endosomal-sorting machinery is independent of the activation status of Gα s . ( a ) In vitro GST pull-down experiment showing that the Gα s activation state did not influence its direct interactions with HRS, dysbindin and GASP-1. In vitro translated 35 S-labelled HRS, dysbindin and GASP-1 were incubated with GST alone or GST–Gα s preloaded with GDP (to mimic the inactive state) or GDP/AlF 4 − or GTPγS (to mimic the active state). Bound proteins were separated by SDS–PAGE and detected by autoradiography. ( b ) GST pull-down experiment in cell lysates demonstrating that the interactions between overexpressed dysbindin, GASP-1 and HRS were independent of the GST–Gα s activation state. Lysates from HEK293 cells transiently transfected with HRS, Myc–dysbindin or Cherry–GASP-1 were incubated with GST alone, inactive GST–Gα s –GDP or active GST–Gα s –GDP/AlF 4 − or GTPγS (as described in a ). Bound proteins were analysed by immunoblotting (IB) for HRS, Myc (dysbindin) and Cherry (GASP-1). The interaction with Gβ1 served as a control to confirm the activation state of GST–Gα s because Gβ1 only binds to inactive Gα s . This control was included in each experiment in a , b . ( c ) The downstream effectors of Gα s were not involved in CXCR4 downregulation. Control and Gα s -depleted HEK293 cells expressing HA–CXCR4 were treated for 8 h with vehicle (DMSO), 10 μM forskolin (an adenylyl cyclase activator) or 10 μM H89 (a PKA inhibitor). The steady-state levels of HA–CXCR4 were analysed by immunoblotting using the indicated antibody. ( d ) Quantification of the HA–CXCR4 levels in c . The data are presented as the percentage of HA–CXCR4 compared with control siRNA cells treated with DMSO. The data are presented as the mean±s.e.m. of ≥3 independent experiments and statistical analysis was performed using the Student’s t- test. ** P ≤0.01. Full size image The signalling-independent role of Gα s in GPCR endosomal sorting was next validated by determining whether the downstream effectors of Gα s altered CXCR4 downregulation. Because Gα s stimulates cyclic AMP production and protein kinase A (PKA) activation, we tested whether forskolin, an adenylate cyclase activator, could rescue Gα s depletion and whether H89, a PKA inhibitor, could mimic Gα s depletion. Control and Gα s -depleted HEK293 cells expressing HA–CXCR4 were treated with vehicle (dimethylsulphoxide (DMSO)), 10 μM forskolin or 10 μM H89 for 8–12 h. CXCR4 abundance was monitored by WB ( Fig. 4c ) and quantified using scanning densitometry to compare multiple independent experiments ( Fig. 4d ). PKA substrates were detected as a positive control for PKA activation ( Fig. 4c ). Although a significant increase in CXCR4 levels was observed in Gα s -depleted cells treated with DMSO, no significant differences were observed between control cells (control siRNA) treated with H89 and vehicle (DMSO) ( Fig. 4d ), indicating that PKA inactivation did not mimic Gα s depletion. Furthermore, no significant differences were observed between Gα s siRNA-treated cells incubated with forskolin or vehicle ( Fig. 4d ), indicating that PKA activation did not rescue the effect of Gα s knockdown on CXCR4 levels, which would be expected if the inhibition of cyclic AMP production in response to Gα s depletion was the cause of the increased CXCR4 levels. We concluded that Gα s activity and its downstream effectors did not play a major role in GPCR endocytic sorting and downregulation. It is increasingly evident that endocytosis has numerous effects on GPCR signal transduction and that GPCR signalling regulates the endocytic machinery. This has blurred the traditional lines separating signalling and endocytosis at both the mechanistic and functional levels. Several proteins have been identified that function in both signalling and endocytosis, the best example being the β-arrestins, which mediate GPCR endocytosis by binding to AP2/clathrin and also participate in signal transduction by scaffolding components of the MAP-kinase pathway [44] , [45] , [46] . The present study determined that Gα s , which is usually involved in GPCR signalling, is a cellular regulator of the post-endocytic sorting of lysosome-targeted GPCRs. This study indicated that Gα s is involved in the regulation of both basal turnover and ligand-mediated degradation of GPCRs. In steady-state cells, Gα s depletion upregulated the expression level of GPCRs that are specifically targeted to lysosomes (CXCR4, DOP, D2R and AT1R). Previous studies have shown that CXCR4 exhibits a high rate of constitutive internalization and turnover [47] , [48] , whereas other GPCRs, such as DOP, have a slow rate of constitutive internalization and turnover [49] . These different turnover rates could explain why Gα s knockdown had a stronger effect on the basal levels of CXCR4. Further analysis of CXCR4 and DOP, which were most affected by Gα s depletion, indicated that Gα s depletion significantly inhibited their lysosomal proteolysis following ligand-stimulated endocytosis without noticeably affecting their internalization and recycling rates. Furthermore, the reduced turnover of CXCR4 and DOP was accompanied by their accumulation on the cell surface and in early endosomes, suggesting a role for Gα s in the trafficking of these GPCRs through the sorting endosomes. The cellular phenotype after Gα s knockdown in this context closely resembled that observed when components of the ESCRT sorting machinery (such as HRS, AMSH and dysbindin) were perturbed [25] , [31] , [50] , implying that Gα s is involved in the endosome-sorting pathway for GPCR trafficking to lysosomes. Indeed, optical imaging demonstrated that Gα s depletion reduced the endosomal sorting of DOP and CXCR4 into the ILVs of MVBs, leading to the accumulation of DOP and CXCR4 on the limiting membranes of early endosomes and preventing receptor downregulation. This work provides the first molecular insight into the mechanism by which Gα s regulates the lysosomal sorting of GPCRs. Our results indicated that Gα s is required in both ubiquitin-dependent and ubiquitin-independent HRS-mediated GPCR sorting, and suggested that Gα s is a scaffold for endosomal-sorting components ( Fig. 5 ). In this study, we determined that Gα s interacts directly with GASP-1 and dysbindin, two accessory sorting proteins that link a subset of GPCRs (such as DOP and D2R) to the HRS component of the ESCRT machinery in an ubiquitin-independent manner. Because the interactions between GASP-1, dysbindin and HRS have been previously reported but not clearly defined [31] , [37] , we further characterized these interactions by showing that dysbindin interacts directly with HRS, but not with GASP-1, and that GASP-1 directly binds to HRS. Moreover, whereas human Gα s was previously shown to directly interact with rat HRS [18] , no interaction was detected between human Gα s and human HRS, suggesting that this interaction is species specific and is indirect in human cells. We propose that Gα s is present on early endosomes, where direct interactions with GASP-1 and dysbindin promote the downstream interaction of a subset of GPCRs with the ESCRT machinery ( Fig. 5a ). These interactions enable the ubiquitin-independent sorting of these GPCRs into the ILVs of MVBs, resulting in lysosomal degradation. This model is supported by the fact that Gα s knockdown had similar effects on DOP and D2R lysosomal sorting and degradation as the knockdown of GASP-1 (refs 30 , 51 , 52 ), dysbindin [31] or HRS [27] ( Supplementary Fig. 1b ). The endosomal sorting role of Gα s was not restricted to GPCRs that interacted with GASP-1 and/or dysbindin. Indeed, the proteolytic downregulation of CXCR4, which is sorted by the ubiquitin- and HRS-mediated ESCRT machinery [25] independent of GASP-1 (ref. 53) [53] and dysbindin ( Supplementary Fig. 1b ), was also affected by Gα s depletion. However, the molecular components of the CXCR4 endosomal-sorting machinery that are regulated by Gα s have yet to be determined ( Fig. 5b ). Current studies are aimed at identifying this cofactor. Interestingly, the downregulation of EGFR, which is also sorted by the ubiquitin-ESCRT machinery, has previously been shown to be altered by Gα s depletion [18] , suggesting that Gα s acts on a general component of the endosomal-sorting machinery for single and seven transmembrane receptors. Future studies should determine whether Gα s influences the downregulation of other GPCRs, such as protease-activated receptor 1 (PAR1), that are sorted to lysosomes independent of ubiquitination, GASP-1 and certain late components of the ESCRT machinery [26] , [54] , [55] . Future studies should also refine our understanding of the role and significance of Gα s in general endosomal sorting. 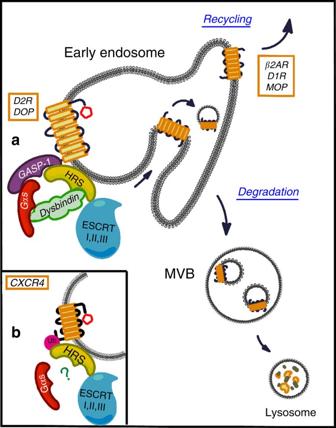Figure 5: Model for Gαsregulation of GPCR endosomal sorting. Gαspromotes the endosomal sorting of GPCRs into the ILVs of MVBs via the ESCRT machinery. (a) Gαsinteracts directly with GASP-1 and dysbindin on endosomal membranes and facilitates/stabilizes their downstream interactions with HRS and the ESCRT machinery. These interactions promote the endosomal sorting and downregulation of a subset of GPCRs, such as DOP and D2R, for which ESCRT sorting is ubiquitination independent. (b) Gαsis also required for the endosomal sorting of GPCRs, such as CXCR4, that are sorted by the ubiquitin- and HRS-mediated ESCRT machinery, but are independent of GASP-1 and dysbindin. However, the molecular components of the Gαs-regulated CXCR4 endosomal-sorting machinery have yet to be identified. Figure 5: Model for Gα s regulation of GPCR endosomal sorting. Gα s promotes the endosomal sorting of GPCRs into the ILVs of MVBs via the ESCRT machinery. ( a ) Gα s interacts directly with GASP-1 and dysbindin on endosomal membranes and facilitates/stabilizes their downstream interactions with HRS and the ESCRT machinery. These interactions promote the endosomal sorting and downregulation of a subset of GPCRs, such as DOP and D2R, for which ESCRT sorting is ubiquitination independent. ( b ) Gα s is also required for the endosomal sorting of GPCRs, such as CXCR4, that are sorted by the ubiquitin- and HRS-mediated ESCRT machinery, but are independent of GASP-1 and dysbindin. However, the molecular components of the Gα s -regulated CXCR4 endosomal-sorting machinery have yet to be identified. Full size image Gα s activity is clearly not limited to the cell surface. Evidence from multiple studies has indicated that Gα s localizes to the endosomes, where it has a functional role in both receptor signalling and trafficking. The presence of Gα s on endosomes has been known for more than a decade, but its role on this intracellular compartment is only beginning to emerge. Gα s is now known to mediate functionally significant signalling from endosomes. Various GPCRs (for example, thyroid stimulating hormone receptor (TSHR), parathyroid hormone receptor, D1R and β2AR) signal via the Gα s -linked activation of adenylyl cyclase directly from the endosome membrane [15] , [20] , [56] , [57] . Moreover, the active forms of β2AR and Gα s have been clearly visualized on endosomes [15] . Gα s has also been implicated in endosomal membrane trafficking functions, such as endosome fusion, pIgR transcytosis and EGFR downregulation [11] , [12] , [13] , [14] , [18] , [19] . An important question is whether the GTPase activity of Gα s is involved in endosomal trafficking. It was previously reported that inactive Gα s interacted with GIV/girdin and was involved in EEA1 membrane recruitment (for EGFR trafficking) [19] , and that the active state of Gα s negatively regulated endosomal fusion [14] . However, in our study, the Gα s activation state did not affect the interactions with the endosomal-sorting machinery (GASP-1, dysbindin and HRS). Consistent with these findings, the effect of Gα s was independent of the Gα s -signalling effectors adenylyl cyclase and PKA, supporting an activation state-independent role for Gα s . These results support a scaffolding, rather than a signalling role for Gα s in GPCR degradation. Interestingly, we noted that none of the GPCRs affected by Gα s depletion are coupled to Gα s for signalling. Indeed, GPCRs coupled to Gα s are sorted to the PM following endocytosis. In fact, we were unable to identify a GPCR coupled to Gα s that is normally sorted to lysosomes. It is possible that the endosomal activation of Gα s by these receptors prevents their interaction with the lysosomal-sorting machinery, or perhaps the Gα s -sorting step occurs later in endosomal maturation, when the recycling GPCRs have already been removed. We intend to investigate these intriguing hypotheses in future studies. The mechanism by which Gα s is translocated to endosomes remains unknown. One possibility is that the activation of a Gα s -linked GPCR stimulates translocation. Following β2AR activation or cholera toxin treatment, Gα s has been shown to dissociate from the PM through activation-induced depalmitoylation of Gα s [58] , [59] , [60] , [61] , [62] . Another possibility is that Gα s is internalized through the endocytic pathway. Following agonist stimulation, Gα s has been shown to localize to vesicles derived from the PM that do not contain β2AR, suggesting that β2AR and Gα s traffic through distinct endocytic pathways [63] , [64] . However, partial colocalization of Gα s with β2AR has been observed on early endosomes [15] , [63] , which corresponds with our data indicating that Gα s colocalizes with DOP or CXCR4 on endosomes. Further studies are necessary to determine whether the stimulation of GPCRs that do not activate Gα s , such as DOP, leads to the translocation of Gα s to the endosomal membrane or whether the stimulation of a Gα s -coupled GPCR increases the translocation of Gα s to endosomes, thereby modulating the lysosomal degradation of other GPCRs. Our findings raise the attractive possibility that Gα s plays a role in both GPCR signalling and trafficking pathways, providing another piece to the intertwining molecular network between these processes. Thus, it is tempting to speculate that Gα s plays a dual role in GPCR signalling via a rapidly responding second-messenger system and via the regulation of GPCR lysosomal trafficking and downregulation. Antibodies and reagents The following antibodies were used in this study: anti-HA monoclonal antibody (mAb) (1:1,000 for WB and 1:500 for IF; Covance, Emeryville, CA, USA), anti-Flag M1 and M2 mAbs and polyclonal antibodies (pAbs) (1:1,000 for WB and 1:500 for IF; Sigma-Aldrich, Saint Louis, MO, USA), anti-Gα s pAb (1:1,000 for WB; Calbiochem, San Diego, CA, USA), anti-HRS mAbs (1:100 for IF; Alexis Biochemicals, San Diego, CA, USA) and pAbs (1:1,000 for WB and 1:100 for IF; Millipore, Billerica, MA, USA), anti-GFP mAbs (1:3,000 for WB and 1:500 for IF; Clontech, Mountain View, CA, USA) and pAbs (1:3,000 for WB and 1:500 for IF; Invitrogen, Carlsbad, CA, USA), anti-EEA1 pAbs (1:1,000 for WB and 1:100 for IF; Thermo Scientific, Rockford, IL, USA), anti-EEA1 goat Abs (1:100 for IF), anti-Gα i 3 and anti-Gβ1 pAbs (1:1,000 for WB) (Santa Cruz Biotechnology, Santa Cruz, CA, USA), anti-CXCR4 (CD184; 1:1,000 for WB; BD Bioscience, Franklin Lakes, NJ, USA) and anti-Myc pAbs (1:2,000 for WB and 1:1,000 for IF; Upstate, Temecula, CA, USA). The anti-dysbindin (1:500 for WB) and anti-GASP-1 (1:10,000 for WB and 1:2,000 for IF) pAbs were generous gifts from Dr Koh-Ichi Nagata (Institute for Developmental Research, Aichi Human Service Center, Japan) and Dr Frédéric Simonin (Université de Strasbourg, France), respectively. DNA constructs pCDNA3.1 vectors expressing either the long (L) or short (S) forms of Gα s were obtained from the Guthrie cDNA Resource Center (Missouri University of Science and Technology, Rolla, MO, USA). The Gα s –GFP fusion protein was a generous gift from Dr Mark Rasenick (University of Illinois, Chicago, IL, USA) and has been previously described [62] . The constitutively active Gα s mutant (Q227L) and constitutively inactive Gα s mutant (G226A, R280K, T284D, I285T and A366S) were generated from Gα s –GFP complementary DNA (cDNA) by QuickChange site-directed mutagenesis as previously described [41] , [42] , [43] . siRNA-resistant forms of the WT, active and inactive Gα s constructs were created by introducing silent substitutions into the Gα s or Gα s –GFP cDNAs within the region of homology to the siRNA Gα s oligo, as previously described [18] . pcDNA3–Gα i3 –YFP has been previously described [65] , and pcDNA3-Gα q and pcDNA3-Gα z were purchased from the Guthrie cDNA Resource Center (Missouri University of Science and Technology) and subcloned into pEGFP-N1. pRK5–Myc–dysbindin was obtained from Dr Koh-Ichi Nagata (Institute for Developmental Research, Aichi Human Service Center, Japan), and untagged dysbindin was generated by subcloning into pcDNA3 and pGEX-KG. pcDNA3–Cherry–GASP-1 and pGEX–GASP-1 were obtained from Dr Frédéric Simonin (Université de Strasbourg, France), and untagged GASP-1 was obtained by subcloning into pcDNA3. pCS2–HRS–RFP was purchased from Addgene (Cambridge, MA, USA), and untagged HRS was subcloned into pcDNA3 and pGEX-KG. pcDNA3–HA–CXCR4 and pcDNA3–HA–β2AR were obtained from Dr Jean-Luc Parent (Université de Sherbrooke, QC, Canada). pcDNA3–Flag–AT1R and pEGFP–C1–DOP were obtained from Dr Richard Leduc and Dr Louis Gendron (Université de Sherbrooke, QC, Canada), respectively. pECFP–C1–CXCR4 was a generous gift from Dr Richard Miller (Northwestern University, Chicago, IL, USA). pcDNA3.1-3*HA–DOP, pcDNA3.1–HA–D1R and pcDNA3.1–HA–D2R were purchased from Missouri S&T, cDNA Resource Center (Missouri University of Science and Technology). Cell culture and transfection COS7 cells were obtained from Dr Klaus Hahn (University of North Carolina, NC, USA), and HEK293T cells were obtained from Dr Alexandra Newton (University of California, San Diego, CA, USA). HEK293 cells stably expressing Flag–DOP or Flag–MOP were obtained from Dr Richard Howells (New Jersey Medical School, Newark, NJ, USA). The cells were grown in Dulbecco’s modified Eagle’s medium (DMEM) high glucose (Invitrogen) containing 10% fetal bovine serum (Hyclone Laboratories, Logan, UT, USA), penicillin and streptomycin. G418 (200 μg ml −1 , Invitrogen) was added to the culture medium for the stable cell lines. Cells were transfected using Lipofectamine 2000 (Invitrogen), X-TremeGENE HP or Fugene 6 (Roche Diagnostic, Indianapolis, IN, USA) according to the manufacturers’ instructions. RNA interference and rescue Scrambled RNA oligos (scramble II duplex) and siRNAs against Gα s (previously described in Zheng et al. [18] ), Gα i3 , Gβ 1 and HRS were purchased from Dharmacon (Lafayette, CO, USA), and dysbindin siRNA was purchased from Qiagen (Hilden, Germany). HEK293T cells were transfected with a final concentration of 100 nM siRNA duplex using Lipofectamine 2000 (Invitrogen) according to the manufacturer’s instructions. The cells were analysed 72 h after the siRNA transfection. The various tagged GPCR cDNAs were transfected using X-tremeGENE HP 48 h before the cell lysis or IF experiments. Rescue experiments were performed by transfecting the cells with cDNAs encoding siRNA-resistant forms of untagged Gα s (short and long) or with control vectors (pcDNA3) using X-tremeGENE HP 10 h after the initial human Gα s siRNA transfection. GPCRs basal expression and degradation assay For the basal expression analysis, HEK293T cells were treated with the Gα s siRNA duplex and transfected with the various tagged GPCRs (as described above). Seventy-two hours after the initial siRNA transfection, all the cells were lysed in RIPA buffer (50 mM Tris-HCl, pH 8, 150 mM NaCl, 1% NP40, 0.1% sodium deoxycholate, 5 mM EDTA and complete protease inhibitors (Roche, Basel, Switzerland)), with the exception of the Flag–DOP and Flag–MOP-stable cell lines, which were lysed in OR buffer (150 mM Tris-HCl, pH 7.5, 300 mM NaCl, 1 mM MgCl 2 , 1 mM CaCl 2 , 1% Triton X-100, 10% glycerol and complete protease inhibitors) as previously described [66] . The lysates were incubated for 1 h at 4 °C and centrifuged at 15,000 g for 20 min at 4 °C. The supernatants were recovered, and the protein concentrations were evaluated by the Bradford assay. Thirty micrograms of each protein sample was aliquoted in Laemmli sample buffer and analysed by immunoblotting. For the degradation assays, HEK cells were treated with the Gα s siRNA duplex and transfected with HA–CXCR4 or HA–DOP (as described above). Forty-eight hours after the initial siRNA treatment, the cells were passaged onto poly- L -lysine-coated six-well plates (Sigma-Aldrich) and grown for an additional 24 h. The cells were washed and incubated with DMEM containing 25 mM Hepes, 0.2% bovine serum albumin (BSA) and 50 μg ml −1 cycloheximide for 15 min at 37 °C. The cells were then incubated with the same medium supplemented with agonist (100 nM SDF1-α or 5 μM DPDPE) for various periods of time. The cells were washed with ice-cold phosphate-buffered saline and lysed in RIPA buffer. The lysates were processed as described above and were analysed by immunoblotting. Cell-surface ELISA Cell-surface ELISAs were performed as previously described [67] . HEK cells were treated with the Gα s siRNA duplex and transfected with HA–CXCR4 or HA–DOP (as described above, 2 μg per P10 dish). Forty-eight hours after the initial siRNA treatment, the cells were plated onto poly- L -lysine-coated 24-well plates (Sigma-Aldrich). After 24 h, the cells were starved for 1 h at 37 °C in DMEM and then incubated with DMEM containing 25 mM Hepes, 0.2% BSA and agonist (100 nM SDF1-α or 5 μM DPDPE) for 30 min or agonist for 30 min followed by antagonist (10 μM Naloxone or AMD3100) for 60 min. The cells were then fixed with 3% formaldehyde, washed with Tris-buffered saline, blocked in 5% BSA and incubated for 1 h with primary antibody (monoclonal anti-HA antibody) and for 45 min with secondary antibody (alkaline phosphatase-conjugated goat anti-mouse antibody; Sigma-Aldrich). The cells were then washed three times, and 250 μl of a colorimetric alkaline phosphatase substrate (diethanolamine and phosphatase substrate; Sigma-Aldrich) was added. The plates were incubated at 37 °C for the appropriate time, and then 250 μl of NaOH (0.4 M) was added to stop the reaction. A 100-μl aliquot of the colorimetric reaction was collected, and the absorbance was measured at 405 nm using a spectrophotometer (Titertek Multiskan MCC/340; Labsystems). Immunoblotting The protein samples were separated on 8 or 10% SDS–polyacrylamide gel electrophoresis (PAGE) gels and transferred to nitrocellulose membranes (Perkin Elmer, Waltham, MA, USA). The membranes were blocked in Tris-buffered saline (20 mM Tris–HCl, pH 7.4, and 150 mM NaCl) containing 0.1% Tween 20 and 5% non-fat dry milk, incubated with primary antibodies for 1 h at room temperature or overnight at 4 °C, subsequently incubated with horseradish peroxidase-conjugated goat anti-rabbit or anti-mouse IgG (Bio-Rad, Hercules, CA, USA) and enhanced using a chemiluminescence detection reagent (Pierce Chemical, Thermo Fisher Scientific, Waltham, MA, USA). Immunofluorescence HEK or COS7 cells were grown on coverslips. Twenty-four to seventy-two hours after transfection, the cells were fixed with 3% paraformaldehyde in 100 mM phosphate buffer, pH 7.4, for 30 min, permeabilized with 0.1% Triton X-100 for 10 min, blocked with 10% fetal bovine serum or goat serum for 30 min, incubated with primary antibodies for 1 h at room temperature and incubated with Alexa Fluor-conjugated secondary antibodies (Molecular Probes, OR). The cells were visualized using an inverted confocal laser scanning microscope (FV1000; Olympus, Tokyo, Japan) equipped with a PlanApo 60x/1.42 oil immersion objective. Olympus FluoView version 1.6a was used to acquire and analyse the images, which were further processed using Adobe Photoshop (Adobe Systems, San Jose, CA, USA). The degree of colocalization between fluorescently labelled GPCRs and the early endosome marker EEA1 was quantified by calculating the Manders coefficient [68] using Olympus FluoView v1.6b colocalization software. The quantitative analysis was performed on 30 size-matched cells for each experimental condition, and the experiments were performed twice. Quantification of DOP–GFP localization in the endosomal lumen HEK cells treated with the control or Gα s siRNA duplex were transfected with DOP–GFP or CXCR4–CFP along with Rab5-Q79L to create enlarged endosomes. Forty-eight hours later, the cells were plated onto poly- L -lysine-coated coverslips and incubated in the presence of 5 μM DPDPE or 100 nM SDF1-α for 90 min before fixation, processing for IF and image acquisition. To quantify the presence of DOP–GFP and CXCR4–CFP in the ILVs of endosomes, measurements were taken from raw data on individual endosomes as previously described [36] , [69] . The quantification was performed on raw data representing confocal cross-sections of individual endosomes. For each endosome, straight-line selections were drawn across the diameter, and pixel intensities across the line were measured. The endosomal diameter was normalized to account for different endosome sizes. The pixel numbers with the first and second maximum pixel intensities, corresponding to pixels on the limiting membrane of the endosome, were normalized to 0 and 100, respectively. The location across the line of pixel 0 was then subtracted from each pixel situated on the line, and this value was divided by the total diameter (in pixels) of the endosome. This generated normalized pixel distances corresponding to the distance across the line occupied by each pixel and was expressed as a percentage. The average background fluorescence was subtracted from the raw pixel intensity values. The pixel intensities for the pixel numbers normalized to 0 and 100 were also normalized to 0 and 100, respectively, generating normalized fluorescence values. The background-corrected pixel intensity values corresponding to pixels that lay 40–60% across the endosomal diameter were averaged, generating a middle-fluorescence value for each endosome. The middle-fluorescence values for multiple cells were compiled, and the mean for each condition is shown. Antibody uptake assay HEK cells were treated with the control or Gα s siRNA duplex and transfected with HA–CXCR4 or HA–DOP (as described above). Forty-eight hours after the initial siRNA treatment, the cells were passaged onto poly- L -lysine-coated coverslips (BD Bioscience) and grown for an additional 24 h. After serum starvation for 1 h, the cells were incubated on ice for 1 h with DMEM containing 25 mM Hepes, 0.2% BSA and anti-HA or anti-Flag (for stable cells) antibody (1:500 dilution). The cells were washed in ice-cold DMEM containing 25 mM Hepes and 0.2% BSA and were incubated at 37 °C with the same medium supplemented with agonist (100 nM SDF1-α or 5 μM DPDPE) for different times. Subsequently, the cells were fixed and processed for IF. To enable the direct comparison of the Flag–DOP or HA–CXCR4 levels remaining in the cells following agonist treatment for different periods of time, all the images within a given experiment were taken with the same magnification and laser intensity settings. Co-immunoprecipitation HEK cells were transiently transfected with GFP or Gα s –GFP together with HRS, Myc–dysbindin or Cherry–GASP-1 cDNA. Forty-eight hours later, the cells were washed twice with ice-cold phosphate-buffered saline, lysed in 50 mM Tris–HCl pH 7.4, containing 150 mM NaCl, 1% NP40 and protease inhibitors for 1 h at 4 °C and centrifuged at 15,000 g for 20 min. The cleared supernatants were incubated with primary antibodies (1 μg of antibody per 1 mg of protein) overnight at 4 °C and then with protein A-Sepharose (GE Healthcare, Piscataway, NJ, USA) or protein G-Sepharose (Zymed, San Francisco, CA, USA) beads for 1 h. The beads were washed three times in lysis buffer and then boiled in Laemmli sample buffer. Bound immune complexes were analysed by SDS–PAGE and immunoblotting. GST pull-down assays GST-fusion proteins were expressed in Escherichia coli BL21 cells and purified on glutathione-Sepharose 4B beads (Pharmacia, Piscataway, NJ, USA) as previously described [70] . The 35 S-labelled in vitro translation products of pcDNA3–dysbindin, pcDNA3–GASP-1 and pcDNA3–HRS were prepared using the TNT T7 rabbit reticulocyte Quick Coupled Transcription/Translation system (Promega, San Luis Obispo, CA, USA) in the presence of [ 35 S]EasyTag EXPRESS labelling mix (73% Met/22% Cys; >1,000 Ci/mmol, Perkin Elmer). A total of 5–10 μg of purified GST or GST-fusion protein was incubated with the in vitro translated products in 20 mM Tris, pH 7.4, 150 mM NaCl, 3 mM EDTA, 0.1% NP40, 1 mM dithiothreitol and complete protease inhibitor for 2 h at 4 °C and washed four times with the same buffer. Bound proteins were eluted with Laemmli buffer, resolved by SDS–PAGE and visualized by autoradiography. For the GST pull-down assays on cell lysates, purified GST-proteins were incubated with 1 mg of lysate from HEK cells expressing Myc–dysbindin, Cherry–GASP-1, untagged HRS or Gα s (S/L) that was prepared as described in the co-immunoprecipitation section. The bound proteins were separated by SDS–PAGE and detected by immunoblotting. In the experiments involving nucleotide loading, GST–Gα s was preincubated with 30 μM GDP alone, 30 μM GDP, 30 μM AlCl 3 and 10 mM NaF (GDP+AlF 4 − ), or 30 μM GTPγS in binding buffer (50 mM Tris-HCl, pH 7.4, 100 mM NaCl, 5 mM EDTA, 0.4% NP40, 2 mM dithiothreitol, 10 mM MgCl 2 and protease inhibitors) for 90 min at room temperature before incubation with in vitro translated proteins or cell lysates. The washing buffer was supplemented with GDP alone, GDP, AlCl 3 and NaF or GTPγs, as during the binding, as previously described [19] , [70] . Bound proteins were either immunoblotted or exposed for autoradiography. Statistical analysis The western blot quantification was performed using Image-Pro Plus Quantification 6.0 software. The GPCR band pixels were normalized to the EEA1 band pixels. Experiments were performed in triplicate, and the results are presented as the mean±s.d. The statistical significance of the differences between the samples was assessed using the Student’s t- test. A value of P <0.05 was considered significant. How to cite this article: Rosciglione, S. et al. Gα s regulates the post-endocytic sorting of G protein-coupled receptors. Nat. Commun. 5:4556 doi: 10.1038/ncomms5556 (2014).